Genome sequence of the model medicinal mushroomGanoderma lucidum Ganoderma lucidum is a widely used medicinal macrofungus in traditional Chinese medicine that creates a diverse set of bioactive compounds. Here we report its 43.3-Mb genome, encoding 16,113 predicted genes, obtained using next-generation sequencing and optical mapping approaches. The sequence analysis reveals an impressive array of genes encoding cytochrome P450s (CYPs), transporters and regulatory proteins that cooperate in secondary metabolism. The genome also encodes one of the richest sets of wood degradation enzymes among all of the sequenced basidiomycetes. In all, 24 physical CYP gene clusters are identified. Moreover, 78 CYP genes are coexpressed with lanosterol synthase, and 16 of these show high similarity to fungal CYPs that specifically hydroxylate testosterone, suggesting their possible roles in triterpenoid biosynthesis. The elucidation of the G. lucidum genome makes this organism a potential model system for the study of secondary metabolic pathways and their regulation in medicinal fungi. Ganoderma lucidum , also known as 'the mushroom of immortality' and 'the symbol of traditional Chinese medicine', is one of the best-known medicinal macrofungi in the world. Its pharmacological activities are widely recognized, as indicated by its inclusion in the American Herbal Pharmacopoeia and Therapeutic Compendium [1] . Modern pharmacological research has demonstrated that G. lucidum exhibits multiple therapeutic activities, including antitumour, antihypertensive, antiviral and immunomodulatory activities [2] . G. lucidum produces a large reservoir of bioactive compounds; thus far, more than 400 different compounds have been identified [3] , making this fungus a virtual cellular 'factory' for biologically useful compounds. Triterpenoids and polysaccharides are the two major categories of pharmacologically active compounds in G. lucidum . In addition to producing these bioactive chemical compounds, G. lucidum , like other white rot basidiomycetes, secretes enzymes that can effectively decompose both cellulose and lignin. Such enzyme activities may prove useful for biomass utilization, fibre bleaching and organo-pollutant degradation [4] . Our understanding of G. lucidum biology is limited despite its venerable role in traditional Chinese medicine and its impressive arsenal of bioactive compounds. Here, we report the complete genome sequence of monokaryotic G. lucidum strain 260125-1, and we identify a large set of genes and potential gene clusters involved in secondary metabolism and its regulation. This genomic information helps elucidate the molecular mechanisms underlying the synthesis of diverse secondary metabolites in medicinal fungi. The genome sequence will make it possible to realize the full potential of G. lucidum as a source of pharmacologically active compounds and industrial enzymes. Genome sequence assembly and annotation We sequenced the genome of the haploid G. lucidum strain 260125-1 ( Supplementary Note 1 and Supplementary Fig. S1 ) using a whole-genome shotgun sequencing strategy. 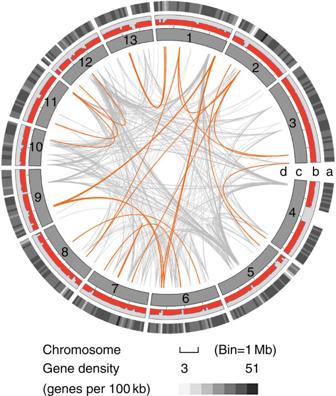Figure 1: An ideogram showing the genomic features ofG. lucidum. (a) GC content was calculated as the percentage of G+C in 100-kb non-overlapping windows. (b) Gene density is represented as the number of genes in 100-kb non-overlapping windows. The intensity of the blue colour correlates with gene density. (c) Pseudochromosome: the diagram represents 13G. lucidumpseudochromosomes. (d) Genome duplication: regions sharing more than 90% sequence similarity over 5 kb are connected by grey lines; those with more than 90% similarity over 10 kb are connected by orange lines (Supplementary Note 6). A 43.3-Mb genome sequence was obtained by assembling approximately 218 million Roche 454 and Illumina reads (~440 X coverage) ( Table 1 and Supplementary Table S1 ). This genome sequence assembly consisted of 82 scaffolds ( Supplementary Table S2 ), which were ordered and oriented onto 13 chromosome-wide optical maps ( Fig. 1 , Supplementary Table S3 and Supplementary Fig. S2 ). A comparison of the sequence scaffolds and optical maps showed greater than 86% congruency, indicating the high quality of the genome sequence assembly. In total, 16,113 gene models were predicted, with an average sequence length of 1,556 bp ( Supplementary Table S4 ), comparable to the genomes of other filamentous fungi [5] , [6] , [7] . On average, each predicted gene contains 4.7 exons, with 85.4% of the genes containing introns. The overall GC content is approximately 55.9% (59.0% for exons, 52.2% for introns and 53.7% for intergenic regions). Repetitive sequences represent approximately 8.15% of the genome. The majority of the repeats are LTR/Gypsy (3.92% of the genome; Supplementary Note 2 and Supplementary Table S5 ). Approximately 70% of the genes were annotated by similarity searches against homologous sequences and protein domains ( Supplementary Table S6 ). Table 1 General features of the G. lucidum genome. Full size table Figure 1: An ideogram showing the genomic features of G. lucidum . ( a ) GC content was calculated as the percentage of G+C in 100-kb non-overlapping windows. ( b ) Gene density is represented as the number of genes in 100-kb non-overlapping windows. The intensity of the blue colour correlates with gene density. ( c ) Pseudochromosome: the diagram represents 13 G. lucidum pseudochromosomes. ( d ) Genome duplication: regions sharing more than 90% sequence similarity over 5 kb are connected by grey lines; those with more than 90% similarity over 10 kb are connected by orange lines ( Supplementary Note 6 ). Full size image Comparisons with other fungal genomes The predicted proteome of G. lucidum was compared with those of 14 other sequenced fungi. OrthoMCL analysis revealed that 4.5% of the predicted proteins in G. lucidum have orthologues in all other species, whereas 43.8% of the proteins are unique to G. lucidum ; approximately 35.3% of the unique proteins have at least one paralogue ( Supplementary Data 1 ). To illuminate the evolutionary history of G. lucidum , a phylogenetic tree was constructed using 296 single-copy orthologous genes conserved in these 15 fungi ( Supplementary Fig. S3 ). The topology of the tree is consistent with the taxonomic classification of these species. The proteome of G. lucidum was also described by the protein family (PFAM) representation ( Supplementary Data 2 and 3 ). The evolution and expansion of single-protein families were examined using CAFÉ [8] . Several protein families were found to have undergone expansion, including families with functions related to anabolism, wood degradation and development ( Supplementary Table S7 ). Noteworthy examples include the expansion of the cytochrome P450 (CYP) family and the major facilitator superfamily (MFS) transporter family. Because these two families have important roles in the biosynthesis and transportation of metabolites, their expansion might well contribute to the diversity of G. lucidum metabolites [9] , [10] . A total of 250 syntenic blocks were identified on the basis of the conserved gene order between G. lucidum and Phanerochaete chrysosporium [11] , corresponding to 3,008 genes and 2,986 genes, respectively, in each genome. On average, each block in the G. lucidum genome includes 12 genes. In all, 92 blocks contain more than ten genes. We also detected 201 collinear blocks common to the G. lucidum and Schizophyllum commune genomes [12] . On average, each block contains 9.92 genes; only 52 blocks have more than ten genes. Several large-scale genomic rearrangements between these fungal species, such as inversions and translocations, were identified, suggesting that extensive genomic rearrangements have occurred since the divergence of these species from their common ancestor ( Supplementary Fig. S4 and Supplementary Note 3 ). Global gene expression analysis RNA-Seq analysis was performed on G. lucidum samples collected at three different developmental stages: mycelia, primordia and fruiting bodies ( Fig. 2a ). The reconstructed transcripts from the RNA-Seq data were mapped to 85% of the predicted G. lucidum genes. As shown in Fig. 2b , 12,646 genes are expressed across all three stages. The ranges of gene expression levels are quite broad during the transitions from mycelia to primordia (T1; left panel, Fig. 2c ) and from primordia to fruiting bodies (T2; right panel, Fig. 2c ). A significant number of genes (4,668) were up- or downregulated during at least one of the stage transitions. During T1, most genes belonging to a particular GO term group demonstrated similar differential expression profiles. Specifically, approximately 20% of these genes are upregulated, and 20% of them are downregulated. However, more than 90% of the genes belonging to the groups related to chromatin assembly (GO: 0006333, GO: 000785 and GO: 0005694) and peroxisome activity (GO: 0005777) are downregulated at T1. During T2, over 90% of the genes involved in intracellular protein transport (GO: 0006886), chromatin assembly or disassembly (GO: 0006333), DNA integration (GO: 0015074) and protein transport (GO: 0015031) are upregulated, reflecting dramatic changes in nuclear structures during this transition ( Supplementary Data 4 ). 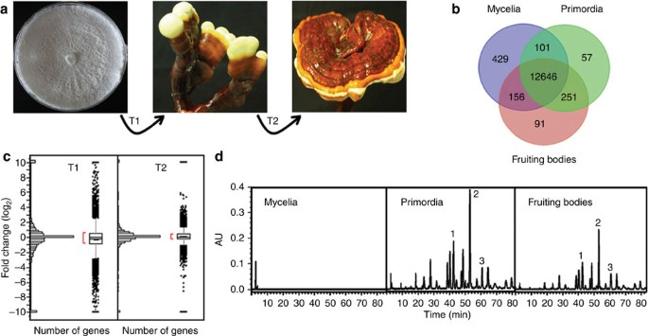Figure 2: Variations in gene expression and triterpenoid content across the developmental stages ofG. lucidum. Samples from each of the three developmental stages were ground in liquid nitrogen. Half of each sample was used for RNA extraction, and the other half was used for chemical profiling. (a) The three developmental stages in the life cycle ofG. lucidum(aerial mycelia of dikaryons, primordia and fruiting bodies) from which samples for gene expression profiling and chemical profiling were collected. (b) Venn diagrams depicting the genes expressed across the different developmental stages. (c) The distribution of gene expression regulation during the stage transitions from mycelia to primordia (T1) and from primordia to fruiting bodies (T2). Thex-axis represents the number of genes, and they-axis represents the log (fold change) for each gene. The distributions of the actual data points are shown on the right sides of panels T1 and T2. The boxes indicate the means (the line in the middle) and the s.d. of the log (fold changes) (from the middle line to the upper and lower edges of the box). (d) HPLC analyses of the triterpenoid contents in the different developmental stages. Three standard compounds are shown: ganoderic acid B (1), ganoderic acid A (2) and ganoderic acid H (3). Figure 2: Variations in gene expression and triterpenoid content across the developmental stages of G. lucidum . Samples from each of the three developmental stages were ground in liquid nitrogen. Half of each sample was used for RNA extraction, and the other half was used for chemical profiling. ( a ) The three developmental stages in the life cycle of G. lucidum (aerial mycelia of dikaryons, primordia and fruiting bodies) from which samples for gene expression profiling and chemical profiling were collected. ( b ) Venn diagrams depicting the genes expressed across the different developmental stages. ( c ) The distribution of gene expression regulation during the stage transitions from mycelia to primordia (T1) and from primordia to fruiting bodies (T2). The x -axis represents the number of genes, and the y -axis represents the log (fold change) for each gene. The distributions of the actual data points are shown on the right sides of panels T1 and T2. The boxes indicate the means (the line in the middle) and the s.d. of the log (fold changes) (from the middle line to the upper and lower edges of the box). ( d ) HPLC analyses of the triterpenoid contents in the different developmental stages. Three standard compounds are shown: ganoderic acid B (1), ganoderic acid A (2) and ganoderic acid H (3). Full size image Triterpenoid biosynthesis Triterpenoids are one of the major groups of therapeutic compounds in G. lucidum , from which more than 150 triterpenoids have been isolated. We observed differences in triterpenoid profiles at different developmental stages. The triterpenoid content was extremely low in cultured mycelia but was markedly increased in the primordia, and it was then clearly reduced during fruiting body formation ( Fig. 2d ). Triterpenoids are synthesized via the mevalonic acid pathway in G. lucidum [13] ( Supplementary Fig. S5 ). The pathway upstream of the cyclization step includes 11 enzymes encoded by 13 genes in G. lucidum . Acetyl-CoA C-acetyltransferases and farnesyl diphosphate synthases are each encoded by two genes in the G. lucidum genome, whereas the remaining nine enzymes are encoded by single-copy genes ( Supplementary Table S8 ). Lanosterol is synthesized by lanosterol synthase (LSS), and it is the common cyclic intermediate of triterpenoids and ergosterol in G. lucidum , from which different metabolic pathways diverge [14] . The steps following cyclization are largely unknown but most likely include a series of oxidation, reduction and acylation reactions. Among these reactions, oxidations catalysed by proteins of the cytochrome P450 superfamily (CYPs) have significant roles in the modification of the lanosterol skeleton ( Supplementary Fig. S5 ). A total of 219 CYP sequences (197 functional genes and 22 pseudogenes) were identified in the G. lucidum genome, and they were classified into 42 families according to standardized CYP nomenclature. When pseudogenes and allelic variants are not considered, G. lucidum has the largest number of CYP genes among all the sequenced fungi. The expression of 197 CYP genes was investigated using real-time PCR. A total of 78 genes were found to be upregulated in the transition from mycelia to primordia and then downregulated in the transition from primordia to fruiting bodies. The expression profiles of these genes were highly correlated with that of LSS (correlation coefficient ( r ) >0.9) ( Fig. 3a and Supplementary Data 5 ). Furthermore, their expression profiles are positively correlated with triterpenoid content profiles during development ( Fig. 2d ), suggesting that some of these 78 CYP genes might be involved in triterpenoid biosynthesis. Of these genes, 28 were classified into novel families unique to G. lucidum , and 38 genes were classified into novel subfamilies of previous known families. The remaining genes belong to subfamilies also found in P. chrysosporium and Postia placenta . On the basis of previous reports on CYPs from P. chrysosporium and P. placenta , we know that some enzymes from the CYP512 and CYP5144 families can only effectively modify an animal steroid hormone, testosterone, from among more than ten potential substrates tested [9] , [15] . Considering the structural similarity of testosterone to the triterpenoids produced by G. lucidum , 15 CYP512 genes and one CYP5144 gene coexpressed with LSS are likely to be involved in triterpenoid biosynthesis ( Fig. 3b and Supplementary Fig. S6 ). The exact roles of these CYPs will be investigated further. 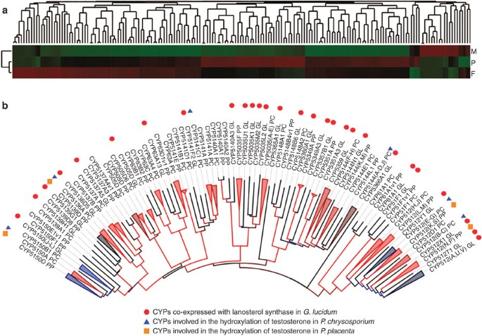Figure 3: CYP gene expression at different developmental stages and phylogenetic analysis coexpressed withLSS. (a) Two-way clustering of gene-expression profiles for the CYP genes expressed across three developmental stages: mycelia (M), primordial (P) and fruiting bodies (F), as quantified by real-time PCR. The relative expression level of each gene was centred on the mean and then unit scaled across the developmental stages. The floor (shown in green) and ceiling (shown in red) of the expression levels were set as twice the s.d. (b) The phylogenetic analysis of CYPs coexpressed withLSSinG. lucidum(GL) and their homologues in Polyporales. A total of 78 coexpressed CYPs from 21 families inG. lucidumand CYPs from the same families inP. placenta(PP) andP. chrysosporium(PC) were included in the tree. The minimal evolution tree was generated with a heuristic search using the Close-Neighbour-Interchange (CNI) algorithm in MEGA (version 5.05). Bootstrap values based on 1,000 replications was set and shown between 50 and 100 just as the branch colours changed from blue, black to red. Moreover, the genes from the same family or subfamily were collapsed and shown as triangles. Figure 3: CYP gene expression at different developmental stages and phylogenetic analysis coexpressed with LSS . ( a ) Two-way clustering of gene-expression profiles for the CYP genes expressed across three developmental stages: mycelia (M), primordial (P) and fruiting bodies (F), as quantified by real-time PCR. The relative expression level of each gene was centred on the mean and then unit scaled across the developmental stages. The floor (shown in green) and ceiling (shown in red) of the expression levels were set as twice the s.d. ( b ) The phylogenetic analysis of CYPs coexpressed with LSS in G. lucidum (GL) and their homologues in Polyporales. A total of 78 coexpressed CYPs from 21 families in G. lucidum and CYPs from the same families in P. placenta (PP) and P. chrysosporium (PC) were included in the tree. The minimal evolution tree was generated with a heuristic search using the Close-Neighbour-Interchange (CNI) algorithm in MEGA (version 5.05). Bootstrap values based on 1,000 replications was set and shown between 50 and 100 just as the branch colours changed from blue, black to red. Moreover, the genes from the same family or subfamily were collapsed and shown as triangles. Full size image In filamentous fungi, evolution has favoured the clustering of genes involved in the biosynthesis of particular secondary metabolites [16] . According to the proposed biosynthetic pathway, at least three CYPs are involved in lanosterol modification in G. lucidum ( Supplementary Fig. S5 ). Therefore, to further characterize the putative gene cluster involved in triterpenoid biosynthesis, we examined the physical clustering of CYP genes in the G. lucidum genome and found 24 clusters containing three or more CYP genes ( Fig. 4 and Supplementary Data 6 ). Of these clusters, two have CYPs that were coexpressed with LSS (average correlation coefficient >0.9). However, ten genes in close proximity to LSS on chromosome 6 did not exhibit strong coexpression with LSS (average correlation coefficient=0.64) ( Supplementary Fig. S7 ), indicating the need for further examination of the organization of the genes involved in triterpenoid biosynthesis in G. lucidum . 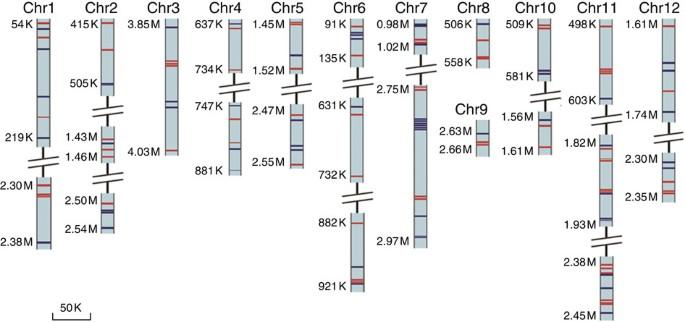Figure 4: Putative CYP gene clusters found in theG. lucidumgenome. The genes are represented by lines on the chromosomal fragments. The colours of the lines indicate whether the genes are in the forward (blue) or reverse (red) orientation. The beginning and end of each cluster is shown to the left, and each cluster is labelled according to the CYP genes it contains. The chromosome numbers are shown at the top. Figure 4: Putative CYP gene clusters found in the G. lucidum genome. The genes are represented by lines on the chromosomal fragments. The colours of the lines indicate whether the genes are in the forward (blue) or reverse (red) orientation. The beginning and end of each cluster is shown to the left, and each cluster is labelled according to the CYP genes it contains. The chromosome numbers are shown at the top. Full size image The biosynthesis of other bioactive compounds in G. lucidum Polysaccharides are another major group of bioactive compounds found in G. lucidum . Among the polysaccharides, the water-soluble 1,3-β-and 1,6-β-glucans are the most active as immunomodulatory compounds [2] , [17] ( Supplementary Fig. S8 ). G. lucidum encodes two 1,3-β-glucan synthases and seven β-glucan biosynthesis-associated proteins containing an SKN1 domain (PF03935); such genes are known to have key roles in the biosynthesis of 1,6-β-glucans in Saccharomyces cerevisiae ( Supplementary Table S9 ). These proteins are well conserved in G. lucidum , S . cerevisiae , P. chrysosporium and P. placenta , suggesting their importance in fungal polysaccharide biosynthesis ( Supplementary Note 4 ) [18] , [19] . LZ-8, the first member of the fungal immunomodulatory protein family, was isolated from G. lucidum in 1989 [20] , [21] . Pharmacological experiments indicated that LZ-8 has anti-tumour and immunomodulation activities [22] , [23] , [24] . All fungal immunomodulatory proteins contain an Fve domain (PF09259.5). Two genes (GL18769 and GL18770) encoding proteins with an Fve domain (PF09259.5) were found in the G. lucidum genome. GL18770 was found to encode a known LZ-8 protein, and GL18769 encodes a protein with 73% identity to LZ-8. The function of GL18769 requires further study. In contrast, no genes encoding Fve domain-containing proteins were found in the P. chrysosporium and P. placenta genomes, suggesting that LZ-8 may be unique to G. lucidum . The G. lucidum genome encodes one non-ribosomal peptide synthase (NRPS) and five polyketide synthase (PKS) genes, including four reducing-type PKSs and one non-reducing-type PKS. Domain analysis indicated these may be functional enzymes ( Supplementary Fig. S9 ). Compared with other fungi, G. lucidum has fewer NRPSs and PKSs, suggesting that G. lucidum may not produce non-ribosomal peptides (NRP) and polyketides (PK) as prolifically as other fungi. Indeed, no NRPs or PKs have been isolated from this species to date; thus, special conditions may be needed to trigger NRPS or PKS gene expression. The terpene synthase family is a mid-sized family responsible for the biosynthesis of monoterpene, sesquiterpene and diterpene backbones [25] . A total of 12 terpene synthase genes were identified in the G. lucidum genome, though triterpenoids are the only type that has been isolated from G. lucidum thus far. Phylogenetic analysis indicated that at least five terpene synthases exhibit high similarity to the characterized terpene synthases from Coprinus cinereus [26] ; these synthases are named Cop1 (germacrene A synthase) (GL22353, 54.5%), Cop2 (germacrene A synthase) (GL25909, 50.3%), Cop3 (γ-muurolene synthase) (GL24515, 65.3%) and Cop4 (γ-cadinene synthase) (GL20244, 55.6%; GL25830, 50.6%) ( Supplementary Fig. S10 ). With the exception of GL22395, all of these genes encode proteins less than 400 amino acids in length and are closely related on the phylogenetic tree, suggesting that all of them may encode sesquiterpene synthases. Some genes encoding tailing enzymes and transporters were found in the vicinity of the PKS, NRPS and terpene synthase genes, suggesting that the biosynthetic gene cluster paradigm may hold true for G. lucidum in the same way that it does in ascomycetes [27] . Recently, more basidiomycete fungi have been sequenced [28] , [29] , [30] , facilitating the understanding of the organization of genes involved in the biosynthesis of secondary metabolites in basidiomycetes. Transporters Transporters have multiple functions, such as the uptake and redistribution of synthesized metabolic end products in the organism, and they are classified into three types: ATP-dependent transporters, ion channels and secondary transporters [31] . A total of 1,063 transport proteins belonging to 134 families were identified in G. lucidum ( Supplementary Data 7 ). Among these transporters, 248 are ATP-dependent transporters, 29 are ion channels and 321 are secondary transporters; the remainder are incompletely characterized transporters. In general, the MFS transporters participate in secondary metabolism, and the ATP-binding cassette (ABC) is involved in the transport of polysaccharides and lipids [32] . In the G. lucidum genome, secondary transporters (321) are the most abundant, with the majority belonging to the MFS family (170), whereas 49 ATP-binding cassette transporters were identified. Some MFS transporters were found in the CYP clusters or other clusters identified using the antiSMASH software [33] , suggesting their possible roles in the biosynthesis of secondary metabolites. Regulation of secondary metabolism Secondary metabolite production and fungal development are regulated in response to environmental conditions. One of the best-known regulatory protein families is the velvet family, and these velvet-domain-containing proteins were also identified in the G. lucidum genome. Two of these proteins, VeA and VelB, are located on the same sequence scaffold. These two proteins interact with the methyltransferase-domain-containing protein LaeA and regulate secondary metabolism and development in Aspergillus . Considering their regulatory roles in previous studies [34] , [35] , we propose a coordinated pathway for secondary metabolism and development in G. lucidum ( Supplementary Fig. S11 ). More than 600 regulatory proteins have been identified in G. lucidum ( Supplementary Data 8 ). A total of 249 predicted regulatory proteins are found in regions that are syntenic with P. chrysosporium or S. commune , implying that part of the gene regulatory network of G. lucidum may be conserved. Zinc-finger-family proteins are reportedly involved in the pathway-specific regulation of fungal secondary metabolites [36] . Among the predicted regulators, 117 CCHC-containing proteins, 81 C2H2-containing proteins and 73 Zn 2 Cys 6 -containing proteins have been identified. Six of these zinc-related proteins were found in clusters predicted using antiSMASH [33] or SMURF [37] ( Supplementary Data 9 and 10 ). Epigenetic modifiers also have important roles in the regulation of secondary metabolism [38] . A total of 33 GCN5-related proteins, 15 PHD-related proteins, 19 SET-related proteins and 8 HDAC-related proteins were identified in the G. lucidum genome. The participation of these predicted proteins in fungal secondary metabolism remains to be experimentally verified. The digestion of wood and other polysaccharides A total of 417 G. lucidum genes could be assigned to carbohydrate-active enzyme (CAZymes) families as defined in the CAZy database [39] ( Supplementary Table S10 ), making this fungus one of the richest basidiomycetes examined so far in terms of the number of CAZymes ( Supplementary Table S11 ). In particular, the genome encodes candidate enzymes for the digestion of the three major classes of plant cell wall polysaccharides: cellulose, hemicelluloses and pectin. Interestingly, although G. lucidum is the richest basidiomycete examined so far in terms of genes encoding enzymes for pectin digestion, its strategy for pectin breakdown relies solely on hydrolytic enzymes; the genome does not encode any pectin/pectate lyases ( Supplementary Data 11 ). In addition, this fungal genome is particularly rich in enzymes that catalyse the decomposition of chitin, with 40 genes assignable to CAZy family GH18, the highest number among known basidiomycetes. Unlike the hydrolysis of polysaccharides, lignin digestion is considered an 'enzymatic combustion' process, involving several oxidoreductases such as laccases, ligninolytic peroxidases and peroxide-generating oxidases [40] . Annotation of the candidate ligninolytic enzymes encoded in the G. lucidum genome revealed a set of 36 ligninolytic oxidoreductases ( Supplementary Table S12 ). Interestingly, compared with model white-rot fungi, such as P. chrysosporium [11] and S. commune [12] ( Supplementary Table S11 ), G. lucidum possesses a large and complete set of ligninolytic peroxidases along with laccases and a cellobiose dehydrogenase. The presence of these enzymes suggests that G. lucidum may exploit different strategies for the breakdown of lignin, including oxidation by hydrogen peroxide in a reaction catalysed by class-II peroxidases. In addition, G. lucidum laccases may degrade recalcitrant lignin compounds in the presence of redox mediators, or they may generate lignocellulose-degrading hydroxyl radicals via Fenton chemistry [41] . In agreement with the presence of candidate class-II peroxidases, several peroxide-generating oxidases were identified in the G. lucidum genome, particularly in the copper-radical oxidase family. Therefore, the distribution of its lignocellulolytic gene families classifies G. lucidum as a particularly versatile white-rot fungus equipped with a remarkable enzymatic arsenal able to degrade all components of wood ( Supplementary Note 5 ). As one of the most famous traditional Chinese medicines, G. lucidum has a long track record of safe use, and many pharmaceutical compounds have been found in this medicinal macrofungus. However, the understanding of the basic biology of G. lucidum is still very limited. Here, we present the genome sequence of G. lucidum generated by next-generation sequencing (NGS) and optical mapping technologies. The high accuracy of the genome sequence was validated using two fosmid sequences obtained by Sanger sequencing technology. With the help of the chromosome-wide optical map for each G. lucidum chromosome, the sequence scaffolds assembled from NGS reads were effectively ordered and oriented onto the optical map scaffolds, which has greatly facilitated the construction of chromosome-wide sequence pseudomolecules. Thus, the combination of optical mapping and NGS represents an effective approach for de novo whole-genome sequencing without cloning or genetic mapping. Our genome sequence analysis revealed a large assortment of genes and gene clusters potentially involved in secondary metabolism and its regulation. In particular, the G. lucidum genome contains one of the richest sets (both in abundance and diversity) of CYP genes known among the sequenced fungal genomes. CYPs generally have important roles in primary and secondary metabolism. Among other Polyporales genomes, P. chrysosporium has 148 CYP genes and 10 CYP pseudogenes in 33 families, and Postia placenta has 186 CYP genes and 5 CYP pseudogenes in 42 families. G. lucidum has 22 families in common with P. chrysosporium and 28 in common with P. placenta . Some of the CYP families are expanded. For example, the CYP512 family has 23 genes in G. lucidum compared with 14 in P. chrysosporium and 14 in P. placenta ( Supplementary Table S13 ). In addition, 11 lineage-specific CYP families were identified in G. lucidum . The expansion of common shared CYP families and the emergence of new CYP families indicate the expansion of the biochemical functions of CYPs in G. lucidum . The discovery of new CYP families seems to accompany the completion of each new fungal genome sequence except in those genomes with unusually small numbers of CYPs. Even among those filamentous fungi that have been highly sampled for sequencing, such as Fusarium and Aspergillus species, newly sequenced genomes continue to reveal novel CYP families. This phenomenon may be due to a larger pool of CYP genes present in a common ancestor, with subsequent gene loss in some species. In addition, lateral gene transfer may occur among fungi. A third possibility involves the evolution of CYPs from an existing family and their rapid divergence accompanied by neofunctionalization [42] . Triterpenoids are a highly diverse group of natural products that are widely distributed in eukaryotes, and many triterpenoids have beneficial properties for human health. To our knowledge, G. lucidum has the most diverse and abundant triterpenoid content of all examined fungi. All triterpenoids isolated from G. lucidum to date are derived from the same lanosterol skeleton. Therefore, the triterpenoid diversity observed in G. lucidum likely originates from different modifications and/or the low substrate specificity of several tailoring enzymes in this pathway. G. lucidum triterpenoids are synthesized via the MVA pathway, which is conserved in all eukaryotes ( Supplementary Fig. S5 ). Compared with the well-studied upstream catalytic steps, little is known about how lanosterol is modified to yield the diverse triterpenoids found in G. lucidum . CYPs have central roles in lanosterol modifications in the proposed triterpenoid biosynthetic pathway. Real-time PCR analysis demonstrated that 78 CYP genes are coexpressed with LSS , suggesting their possible roles in triterpenoid biosynthesis. Recently, a comprehensive functional analysis of CYPs from P. chrysosporium and P. placenta was carried out using a wide variety of compounds as substrates [9] , [15] . Interestingly, we found that multiple CYPs can catalyse the hydroxylation of testosterone, suggesting that their natural substrates are structurally related to the steroids. These CYPs include CYP512 (C1, E1, F1, G2), CYP5136 (A1, A3), CYP5141C1, CYP5144J1, CYP5147A3 and CYP5150A2 in P. chrysosporium and CYP512 (N6, P1, P2), CYP5139D2 and CYP5150D1 in P. placenta . However, of these CYPs, CYP5136 (A1, A3), CYP5141C1, CYP5147A3, CYP5150 (A2, D1) and CYP5139D2 show low substrate specificity, as they can effectively modify several other compounds, such as biphenyl, carbazole and so on. Therefore, these enzymes are less likely to use steroids as their natural substrates. In contrast, the enzymes from the CYP512 and CYP5144 families are most likely involved in steroid modification in the two species. In G. lucidum , we found 15 genes from the CYP512 family and one gene from the CYP5144 family that are coexpressed with LSS ( Supplementary Fig. S6 ). On the basis of structural similarities between steroids and the G. lucidum triterpenoids, these enzymes are more likely to catalyse hydroxylation reactions on the cyclic skeletons of the triterpenoids in G. lucidum . Interestingly, in addition to the genes involved in the biosynthesis of triterpenoids and polysaccharides, we found genes that may be involved in the biosynthesis of NRPs, PKs and other kinds of terpenes. These compounds have not previously been isolated from G. lucidum , suggesting that their synthesis might be tightly regulated. This example shows that genome analyses can provide insight into the complete chemical profile of an organism. Some of the synthetic pathways encoded in this genome might contribute to the therapeutic activities of G. lucidum . In summary, the elucidation of the G. lucidum genome makes it a compelling model system for studying the biosynthesis of the pharmacologically active compounds produced by medicinal fungi. The identification of numerous lignin degradation enzymes will accelerate the discovery of complete lignin degradation pathways necessary for the strategic exploitation of these enzymes in industrial settings. Therefore, the comprehensive understanding of the G. lucidum genome will pave the way for its future roles in pharmacological and industrial applications. Strain and culture conditions G. lucidum is a species complex that shows tremendous intra-species diversity [43] . The G. lucidum dikaryotic strain CGMCC5.0026, belonging to the G. lucidum Asian group, was obtained from the China General Microbiological Culture Collection Center (Beijing, China) and is one of the most widely used isolates for the production of G. lucidum medicinal material in China. The monokaryotic strain G.260125-1 used for whole-genome sequencing was derived from the strain CGMCC5.0026 by protoplasting. Vegetative mycelia were grown on potato dextrose medium in the dark at 28 °C. Liquid cultures were shaken at 50 r.p.m. The primordia and fruiting bodies of the strain CGMCC5.0026 used for transcriptomic analyses were cultivated on Quercus variabilis Blume logs at HuiTao Pharmaceutical Company (LuoTian, Hubei Province, China). All strains are available on request. Construction of an optical map Protoplasts of the monokaryotic strain G.260125-1 were collected by centrifugation at 1,000 g for 10 min −1 and were then diluted to a final concentration of 2×10 9 cells ml −1 . A solution of 1.2% low-melting-point agarose in 0.125 M EDTA (pH 7.5) was heated to 45 °C in a water bath and was then added to the protoplast suspension. The mixture was pipetted thoroughly using a wide-bore tip and was then placed at 4 °C to solidify. The solidified gel was sliced into pieces and incubated in 50 ml of digestion buffer (0.5 M EDTA, 7.5% β-mercaptoethanol) at 37 °C overnight. Then, the buffer was replaced with NDSK buffer (0.5 M EDTA, 1% (v/v) N-lauroylsarcosine, 1 mg ml −1 proteinase K) [44] . DNA samples for optical mapping were obtained by melting DNA gel inserts at 70 °C for 7 min, and then digesting with β-agarase (New England Biolabs, USA) at 42 °C for 2 h. The optimal concentration for mapping was determined by performing serial dilutions in TE buffer, and wide-bore pipette tips were used for the liquid transfers. T7 DNA (Yorkshire Bioscience, UK) at a concentration of 30 pg μl −1 was added to TE and mixed by pipetting up and down using a wide-bore pipette tip before the addition of genomic DNA. DNA solutions were loaded into the silastic microchannel device, and the DNA molecules were stretched and mounted onto the optical mapping surfaces through capillary action and the electrostatic binding of DNA molecules to the positively charged optical mapping surfaces. Mounted DNA molecules were digested by the restriction endonuclease Spe I in NEB Buffer 2 (50 mM NaCl, 10 mM Tris–HCl, 10 mM MgCl 2 , 1 mM dithiothreitol, pH 7.9; New England Biolabs) without BSA, and Triton X-100 was added to the digested DNA at a final concentration of 0.02%. Digested DNA molecules were then stained with 12 μl of 0.2 μM YOYO-1 solution (5% YOYO-1 in TE containing 20% β-mercaptoethanol; Eugene, USA). Fully automated imaging workstations were used to generate single-molecule optical data sets for whole-genome map construction. Genome sequencing and assembly The genomic DNA of G. lucidum was sequenced using the Roche 454 GS FLX (Roche, USA) and Illumina GAII (Illumina, USA) NGS platforms. Following pre-processing, the Roche 454 reads were assembled into a primary assembly using CABOG [45] and then scaffolded with Illumina paired-end and mate-pair reads using SSPACE version 1.1 [46] . Finally, the short reads were subjected to error correction and gap filling using Nesoni (version 0.49) and SOAP GapCloser [47] , respectively. The finished chromosome-wide sequence pseudomolecules were constructed by anchoring and orienting the final sequence scaffolds onto the whole genome physical maps of G. lucidum generated by an optical mapping system [48] , [49] . Gene prediction and annotation Gene models were predicted using the MAKER pipeline [50] . The repeat sequences were masked throughout the genome using RepeatMasker (version 3.2.9) and the RepBase library (version 16.08). Gene structures were predicted with a combination of ab initio Fgenesh [51] , [52] , SNAP [53] and Augustus [54] ; comparisons with protein sequences were performed using BLASTX and exonerate: protein2genome. In parallel, comparisons with Roche 454 EST sequences were performed using BLASTN and exonerate: est2genome against a set of Roche 454 EST contigs from three different developmental phases: mycelia, primordia and fruiting bodies. A set of 16,113 predicted gene models were obtained, and more than 1,600 genes were manually curated using Apollo software. All of the predicted gene models were functionally annotated by their sequence similarity to genes and proteins in the NCBI nucleotide (Nt), non-redundant and UniProt/Swiss-Prot protein databases. The gene models were also annotated by their protein domains using InterProScan. All genes were classified according to Gene Ontology (GO), eukaryotic orthologous groups and KEGG metabolic pathways. Repeat content The REPET package (version 1.4) [55] , [56] was used to detect and annotate transposable elements in G. lucidum . Satellites, simple repeats and low-complexity sequences were annotated separately using RepeatMasker. Transcriptome sequencing and analyses For the Roche 454 sequencing, complementary DNA was synthesized using SMART technology as previously described [57] and sequenced using the standard GS FLX Titanium RL sequencing protocol (Roche). The Roche 454 reads were assembled using the GS De Novo Assembler (version 2.5.3). An RNA-Seq analysis was performed according to the protocol recommended by the manufacturer (Illumina). The reads from different phases were mapped to the whole-genome assembly using BLAT (version 0.33) [58] with the following settings: 90% minimum identity and 100-bp max intron length. The statistical models for maximum likelihood and maximum a posteriori implemented in Cufflinks (version 1.1.0) were used for expression quantification and differential analysis [59] . The abundances are reported as normalized fragments per kb of transcript per million mapped reads. A gene is considered significantly differentially expressed if its expression differs between any two samples from the three stages with a fold change >2 and a P -value <0.05 as calculated by Cufflinks. Quantitative PCR Following digestion with DNase, the total RNA was reverse transcribed into single-stranded complementary DNA. Quantitative PCR was performed three times for each sample using SYBR green (Life Technologies, USA) on an ABI PRISM 7500 Real-Time PCR System (Life Technologies). The expression data for the CYPs were normalized against an internal reference gene, glyceraldehyde-3-phosphate dehydrogenase ( GAPDH ). The relative expression levels were calculated by comparing the cycle threshold (Ct) of each target gene with the 'housekeeping' gene GAPDH using the 2 −ΔΔCt method. CYP annotation and analysis The reference CYP sequences were downloaded from http://drnelson.uthsc.edu/P450seqs.dbs.html . All predicted proteins were then used to search the reference CYP data set using the BLASTP program with a cutoff E-value <1e−5. The selected proteins were manually curated and named according to the standard sequence homology criteria for CYP nomenclature. A physical CYP gene cluster was defined as three or more CYPs present within a 100-kb sliding window of the genomic sequence or fewer than 10 genes between CYPs after they had been sorted into groups along the chromosomes. If two adjacent clusters overlapped, they were merged to form one larger cluster [60] . Carbohydrate-active enzyme annotation All putative G. lucidum proteins were searched against entries in the CAZy [39] database using BLAST. The proteins with e-values smaller than 0.1 were further screened by a combination of BLAST searches against individual protein modules belonging to the GH, GT, PL, CE and CBM classes, and CBM and HMMer (version 3.0) were used to query against a collection of custom-made hidden Markov model (HMM) profiles constructed for each CAZy family. All identified proteins were then manually curated. Lignin digestion enzyme annotation HMM profiles were constructed for each family of lignin-digesting enzymes and were used to classify G. lucidum genes into sequence-based families, termed AA1 to AA8 (Levasseur and Henrissat, unpublished data). All identified proteins were then manually curated. Data availability More detailed descriptions of the methods are provided in Supplementary Methods. All of the data generated in this project, including those related to genome assembly, gene prediction, gene functional annotations and transcriptomic data, may be downloaded from our interactive web portal at http://www.herbalgenomics.org/galu . S.C. initiated the G. lucidum genome project; S.C., C.S. and C.Liu designed and coordinated the project; J.X., C.Li., L.W., X.G. and J.Q. sequenced the genome; S.Z. and D.C.S. performed the optical mapping; Y.Z. and Y.L. assembled the genome; Y.Z. and C.Liu coordinated the annotation process; D.R.N., J.X., X.L., L.S., L.H., L.X., X.X., Y.N., Q.L., H.Y., J.Z. and H.C. annotated and curated the genes; Y.S., H.L., Z.W. and M.L. performed the experiments; J.S., D.R.N., B.H., A. Levasseur, M.V.H. and A. Lv. interpreted the experiments; C.S., C.Liu, J.S., J.X., Y.J., B.H., A. Levasseur and D.R.N. wrote the paper; S.C. and J.S. coordinated the writing of the paper. Accession codes: This whole-genome sequencing project has been deposited at Genome under the project accession number PRJNA71455. Sequence reads have been deposited in the short-read archive at GenBank under the following accession numbers: SRA043914 contains the Roche 454-generated genomic reads, SRA048014 contains the Illumina GA-generated genomic data, SRA048974 contains the Roche 454-generated transcriptome reads and SRA048015 contains the Illumina RNA-Seq reads. How to cite this article: Chen, S. et al . Genome sequence of the model medicinal mushroom Ganoderma lucidum . Nat. Commun. 3:913 doi: 10.1038/ncomms1923 (2012).